Observation and theory of X-ray mirages The advent of X-ray lasers allowed the realization of compact coherent soft X-ray sources, thus opening the way to a wide range of applications. Here we report the observation of unexpected concentric rings in the far-field beam profile at the output of a two-stage plasma-based X-ray laser, which can be considered as the first manifestation of a mirage phenomenon in X-rays. We have developed a method of solving the Maxwell–Bloch equations for this problem, and find that the experimentally observed phenomenon is due to the emergence of X-ray mirages in the plasma amplifier, appearing as phase-matched coherent virtual point sources. The obtained results bring a new insight into the physical nature of amplification of X-ray radiation in laser-induced plasma amplifiers and open additional opportunities for X-ray plasma diagnostics and extreme ultraviolet lithography. The role of X-rays in the modern world is quite significant not only from a scientific point of view but also because of their practical use [1] . An obvious example is the prominent contribution of X-rays in medicine and for deciphering the structure of macromolecules, including DNA. After the realization of X-ray lasers, the studies that use X-rays have reached a qualitatively new level [2] , [3] , [4] , and a new era in the development of X-ray physics was opened by the advent of laboratory X-ray lasers [5] , [6] , especially ‘desktop’ X-ray lasers, such as transient collisional excitation lasers [7] , [8] , [9] , [10] , its grazing-incidence pumped scheme (GRIP) modification scheme [11] , [12] , optical-field-ionization collisional-excitation lasers [13] and the capillary discharge plasma lasers [14] , [15] . High-order harmonics [16] , [17] , [18] , [19] , [20] , used as a ‘seeded beam’ in plasma-media X-ray lasers [21] , [22] , [23] , [24] and X-ray free-electron lasers [25] , as well as the two-stage transient-collisional excitation oscillator-amplifier scheme [26] , [27] , allowed to improve coherent properties of X-ray lasers [28] , [29] , [30] . However, the coherence of output radiation of modern X-ray lasers is far from perfection [31] , and efforts of many scientific groups are aimed at improving both the temporal and spatial coherence of X-ray lasers. Here we report the observation of an unknown interference structure in the spatial profile of the output beam of a two-stage plasma-media X-ray laser. After theoretical analysis, we have reached an understanding of this new X-ray mirage mechanism that can drastically influence the spatial characteristics of X-ray laser beams. Experimental observation of X-ray mirages The experiment with the soft X-ray laser (SXRL) facility has been performed at Kansai Photon Science Institute of Japan Atomic Energy Agency. The experimental setup is shown in Fig. 1 and is briefly described in the Methods section. We have found the appearance of the interference pattern in the form of concentric rings in the cross-section of the beam at the output of the two-stage X-ray plasma laser. The appearance of such interference pattern in the spatial profile of the output beam is rather unexpected observation, because there is no apparent physical causes that can lead to it. Moreover, to our knowledge, nothing like this has previously been observed not only in X-rays but also in the visible range. 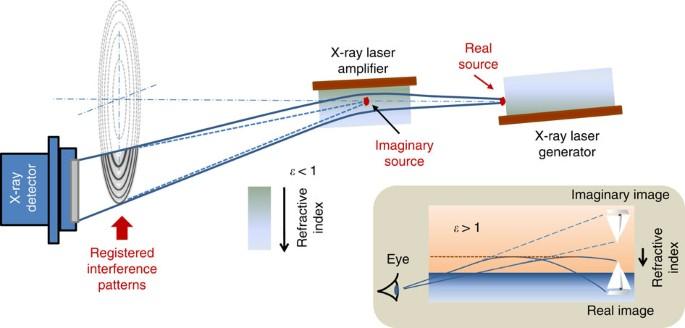Figure 1: Scheme of the X-ray mirage observation. The X-ray mirage appears as a circular interference pattern. The centre of interference rings is located on the axis passing through two coherent sources: the real source created by the X-ray laser generator and the imaginary source formed by X-ray plasma amplifier. Inset: origin of an optical mirage in the earth atmosphere. Figure 1: Scheme of the X-ray mirage observation. The X-ray mirage appears as a circular interference pattern. The centre of interference rings is located on the axis passing through two coherent sources: the real source created by the X-ray laser generator and the imaginary source formed by X-ray plasma amplifier. Inset: origin of an optical mirage in the earth atmosphere. Full size image Spatial-intensity distribution of an output beam of the two-stage SXRL obtained in a single shot at the distance of 3,314 mm from the amplifier is shown in Fig. 2a . The profile of X-ray beam was recorded by a back-illuminated X-ray CCD (charge-coupled device) (Princeton Inc.) with 2,048 × 2,048 pixels of a 13.5-μm pixel size. The narrow vertical dark stripe on the left edge of the image is a shadow of the amplifier target. The bright spot elongated in the horizontal direction is a footprint of output amplified radiation. Intensity distributions for two regions of the beam are shown in the insets together with their horizontal traces. The ring structure is clearly observed in the spatial distribution of the beam, almost over a whole-beam profile. The ring structures were recorded consistently from shot to shot. It was found that the ring structure exists at relative delays of ≤10 ps and for angles between oscillator and amplifier targets ≤0.6°. Interference fringes were observed only in the two-stage laser operation mode, that is, when the generator and amplifier were turned on simultaneously. 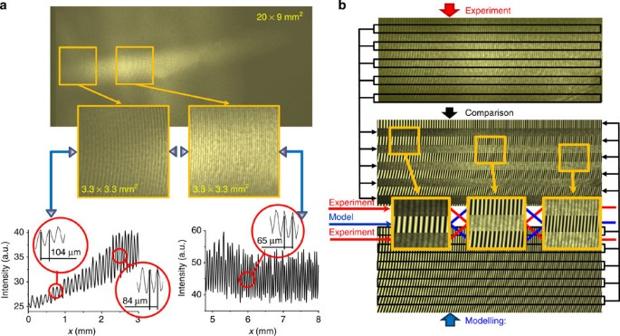Figure 2: X-ray mirage interference patterns. (a) Interference pattern recorded by CCD camera in a single laser shot in the far-field beam profile at the distance of 3,314 mm from the amlifier. Traces show the decrease of the interference fringes period with increasing the distance from the amplifier target. (b) Enlarged central bright part of the experimental image (top); calculated interference pattern from two coherent point sources located at the distance of 203 mm between them (bottom); comparison between theory and experiment by combining of images as indicated by black arrows (centre); in the enlarged fragments of the central image, red and blue arrows show which of the bands refer to the theory and which to the experiment. Figure 2: X-ray mirage interference patterns. ( a ) Interference pattern recorded by CCD camera in a single laser shot in the far-field beam profile at the distance of 3,314 mm from the amlifier. Traces show the decrease of the interference fringes period with increasing the distance from the amplifier target. ( b ) Enlarged central bright part of the experimental image (top); calculated interference pattern from two coherent point sources located at the distance of 203 mm between them (bottom); comparison between theory and experiment by combining of images as indicated by black arrows (centre); in the enlarged fragments of the central image, red and blue arrows show which of the bands refer to the theory and which to the experiment. Full size image Additional series of experiments were undertaken, where a LiF crystal [32] was used for recording the spatial-intensity distribution of the X-ray laser beam averaged over 30 laser shots. The measurements indicate high stability of the interference patterns, leading to the conclusion that the phenomenon has a fundamental character, it does not depend on fluctuating plasma parameters and that both sources are rigidly phased. First of all, we suggested that detected rings are produced by an interference of radiation emitted by two coherent point sources. The first source is evident. It is formed by the oscillator. We could determine relative position of the second source by matching the experimentally observed interference pattern with the calculated one. For comparison, we selected an area of 7.3 × 2.8 mm 2 in the centre of the beam profile shown in Fig. 2a . The result of comparison of the experimentally obtained interference pattern with the numerically calculated pattern is shown in Fig. 2b . The horizontal rectangle grids were superimposed on the images to facilitate a comparison. It is evident that there is nearly perfect agreement between the experimental and calculated interference fringes. The distance between the sources determined by this method has turned out to be 203±2 mm. Because of the rather low spatial coherence of the generator radiation and related spotty near-field beam structure, it can be concluded that the first of the interfering sources should be located near the exit surface of the plasma generator. Considering that lengths of both generator and amplifier plasmas are ~6 mm, the distance between their centres is ~206 mm and the distance between sources is ~203 mm, we come to the conclusion that the second virtual source should be located somewhere in the middle of the plasma amplifier. Theory of X-ray mirages in laser-induced plasma The results of the previous section indicate that the output beam can be treated as formed by radiation of two coherent almost ideal point sources, which are in phase with each other. The first, real source, is located inside the oscillator, and the second—virtual imaginary source—is inside the amplifier. The appearance of a coherent imaginary source cannot be explained by nonlinearity of the absorption process of individual particles homogeneously dispersed in space. In such a model, the phase front of the stimulated emission should repeat the phase front of an initial wave and, therefore, could not create a spherical wave with a phase front of another curvature. However, another approach turned out to be productive. As it is known, laser-induced plasma has unique electrodynamic properties. We suggested that because of its high density and strong localization in space, such a plasma may provide conditions for X-ray mirage creation similar to formation of mirages, which are observed in the inhomogeneously heated earth atmosphere ( Fig. 1 inset). According to the proposed hypothesis, we have developed the optical theory of X-ray mirage formation in extended optically inhomogeneous amplifying medium. The mirage is a structure that is formed in space. Therefore, we can restrict ourselves to the study of a spatial behaviour of radiation and cannot be interested in the temporal dynamics of the amplified pulses [33] . Suppose that the wide divergent X-ray beam incidents on a small piece of such medium, in particular, on a plasma clot ( Fig. 3a ). Several factors will influence the formation of a mirage. Not only the spatial distribution of the refractive index but also a gain of the medium will have a significant role in the process. Besides, as in typical X-ray lasers the gain coefficient is very high, it is necessary to consider the effects of saturation in signal amplification. 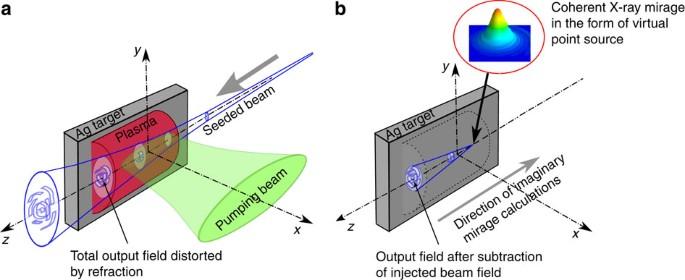Figure 3: Plasma as an optical inhomogeneous medium capable of producing X-ray mirages. (a) Emergence of the distorted radiation during propagation of a seeded X-ray beam through inhomogeneous plasma according to Equation 2. (b) Scheme illustrating the idea of X-ray mirage calculation according to Equation 3. Figure 3: Plasma as an optical inhomogeneous medium capable of producing X-ray mirages. ( a ) Emergence of the distorted radiation during propagation of a seeded X-ray beam through inhomogeneous plasma according to Equation 2. ( b ) Scheme illustrating the idea of X-ray mirage calculation according to Equation 3. Full size image Within the formulated problem, the beam propagation in an extended optically inhomogeneous amplifying medium can be described by the wave equation, which can be rewritten in the paraxial approximation for slowly varying amplitudes E ( x , y , z , t )=1/2{ A ( x , y , z ) e i ( ωt − kz ) + c.c. } as: where A ( x , y , z ) is a complex amplitude of the X-ray electric field, propagating in z direction; ε ( x , y , z ) is the dielectric permittivity of a medium at the frequency ω , the imaginary part of which models the gain. For describing the interactions of X-rays with the amplifying plasma, it is enough to use the semi-classical approximation, which leads to a self-consistent system of the Maxwell–Bloch equations [31] , [33] , consisting of the Maxwell’s wave equation (equation (1) in our case) and the constitutive equations describing the dynamics of a two-level medium. In our model, equation (1) is written for Fourier components of the field at the frequency ω . As it is known, in the Fourier representation constitutive equations become independent on time. As a result, the amplifying medium can be described by the effective dielectric permittivity (see, for example, Dorofeenko et al . [34] ). If the radiation frequency coincides with the transition frequency, as in the case of amplification of X-ray radiation in the plasma, the effective dielectric permittivity can be written as ε ( x , y , z )=1− . Here n e ( x , y , z ) is the electron density of the plasma; n c is the critical electron density of the plasma; G ( x , y , z )= G 0 g ( x , y , z ) is a small-signal gain distribution; x , y , z are Cartesian coordinates; λ is the wavelength; and β is the parameter characterizing the gain saturation, which depends on an off-diagonal element of the transition dipole moment and on the characteristic relaxation times for polarization and population inversion. The form of the real part of ε was chosen in accordance with the data presented in Gasparyan et al . [35] In numerical calculations, we shall also consider the plasma is uniform along z axis. The last assumption means that the functions n e ( x , y ) and G ( x , y ) depend only on x , y and do not depend on z . We also assume that x axis is perpendicular to the target surface and y axis is parallel to the target surface. We use the term ‘X-ray mirage’ in the same sense as it is understood in the optical range. Mathematically, this is a part of the total radiation that remains after subtracting from it the initial radiation under the assumption that the initial radiation propagates through a medium without distortion due to inhomogeneity of a medium. According to this definition, we can represent the amplitude A ( x , y , z ) as the sum of two terms A ( x , y , z )= A inc ( x , y , z )+ A M ( x , y , z ), where A inc ( x , y , z ) is the amplitude of an incident beam propagating in empty space and A M ( x , y , z ) is the amplitude of the mirage radiation emerging in the plasma. Substituting A ( x , y , z ) into equation (1), we can find that A M ( x , y , z ) satisfies the equation: which can be regarded as an equation for the complex amplitude of X-ray mirages. To determine what imaginary source corresponds to the output mirage radiation A M ( x , y , L ), as well as to determine its position and shape, it is enough to ‘run’ the output radiation back in the geometry where the plasma is removed ( Fig. 3b ). To do this, taking into account the symmetry of the wave equation with respect to time reversal, it is sufficient to solve the equation: with the initial condition ( x , y ,0)= A M ( x , y , z L ), where ( x , y , z ) is the complex amplitude of an imaginary source; Z L is the coordinate of the exit face of plasma. For numerical calculations, we will choose the origin of the Cartesian coordinate system on the input surface of the plasma and will consider that in the x − y plane it coincides with the maximum of the gain distribution. Our numerical simulations show that in a typical laser-induced plasma used in X-ray lasers, a coherent mirage in the form of an imaginary point source can arise. For our laser geometry, the position of this point source in space is in accordance with obtained experimental data. As a plasma is the inhomogeneous extended medium, it is obvious that the wave front of an amplified beam is distorted due to refraction ( Fig. 3a ). To find a total field at the exit of the plasma, we should solve equation (2). However, to talk about a mirage, and, moreover, about a coherent mirage, we should be able to treat the additional radiation arising in the plasma as the radiation emitted by an imaginary source with clearly defined form in space. In accordance with the proposed mechanism, we can state that X-ray mirage in the form of a coherent virtual point source will be observed in the plasma amplifier if four following conditions are satisfied: (1) there is a local maximum in n e ( x , y ) distribution, (2) spatial location of a G ( x , y ) region coincides with the position of the local maximum of n e ( x , y ), (3) spatial size of a gain region is equal or less than the width of the n e ( x , y ) local maximum and (4) uniformity of the plasma along the direction of beam propagation is sufficiently high. All conditions are not unique for the plasma induced by short laser pulses on the surface of solid targets [36] , [37] , [38] . The additional comments are presented in Supplementary Discussion . Results of the hydrodynamic calculations [36] , [37] , [38] show that the conditions (1) and (2) of the mirage emergence do not always exist in the plasma. These conditions are realized only at a certain stage of its temporal evolution as can be seen from Fig. 4a and Supplementary Fig. S1 . This explains the fact that in our experiments the mirage disappeared when the delay between the pumping laser pulses that initiated the plasma generator and the plasma amplifier exceeded 10 ps. We believe that disappearance of the mirage at angles >0.6° happens mainly because of violation of the condition (4). 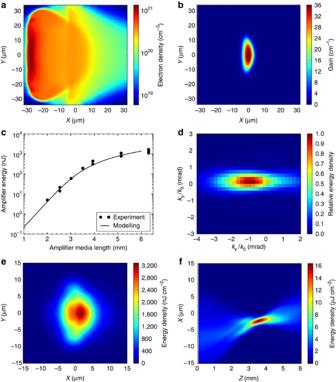Figure 4: Results of the numerical simulations of X-ray mirages. (a,b) Spatial profiles of the electron densityne(x,y) and small-signal gainG(x,y), which were used for plasma modelling. Data are based on the results of two-dimensional hydrodynamic plasma model presented in Berrillet al.37(c) Output energy of the amplified seeded beam versus the amplifier medium length: results of our numerical simulation are shown as the solid curve and the dark circles that demonstrate the experimentally measured output energy of our X-ray amplifier26. (d) Calculated angular spectrum of the output X-ray radiation. (e) Intensity distribution of X-ray mirage radiation at the output of the amplifier. (f) Intensity distribution of X-ray mirage radiation in the vicinity of its imaginary waist. Figure 4: Results of the numerical simulations of X-ray mirages. ( a , b ) Spatial profiles of the electron density n e ( x , y ) and small-signal gain G ( x , y ), which were used for plasma modelling. Data are based on the results of two-dimensional hydrodynamic plasma model presented in Berrill et al . [37] ( c ) Output energy of the amplified seeded beam versus the amplifier medium length: results of our numerical simulation are shown as the solid curve and the dark circles that demonstrate the experimentally measured output energy of our X-ray amplifier [26] . ( d ) Calculated angular spectrum of the output X-ray radiation. ( e ) Intensity distribution of X-ray mirage radiation at the output of the amplifier. ( f ) Intensity distribution of X-ray mirage radiation in the vicinity of its imaginary waist. Full size image The above arguments imply that only the region near the local maximum of n e ( x , y ) surface is essential for X-ray mirage formation. The shape of the density profile n e ( x , y ) outside the local maximum has almost no effect on the result. The position of the virtual source is mainly determined by the curvature of the n e ( x , y ) surface at its maximum, that is, by second derivatives with respect to x and y . If they are not equal, the astigmatic virtual source is formed. In the case of weak diffraction, the position of an imaginary source can be analytically calculated in the ray-tracing approximation. In this approximation, the position of an imaginary source is very sensitive to the width Δ ed of a n e ( x , y ) local maximum; more accurately, it is proportional to the square of this width. The spatial distribution of the gain G ( x , y ) also affects the properties of the source, but in a different way. Width of the local maximum at G ( x , y ) surface defines the size of a source in its imaginary focus and, therefore, determines the diffraction divergence of mirage radiation. In the case of asymmetric G ( x , y ) surface in the vicinity of a local maximum, the size of a virtual point source will be different in x and y directions, leading to a different beam divergence over these coordinates. The results of calculations showing the formation of a mirage for a rather large size of the gain area, when we can neglect the diffraction effects, are shown in Supplementary Fig. S2 and Supplementary Movie 1 . For a small size of gain area, diffraction effects begin to have a significant role. Equation (2) naturally takes into consideration the diffraction effects, but, unfortunately, in the conditions of strong diffraction, it is impossible to give a simple picture of mirage formation, and the numerical solution of equation (2) is required. To calculate a mirage according to equations (2 and 3), we need to know the functions n e ( x , y ) and G ( x , y ). Because these functions cannot be measured experimentally, we used the results of hydrodynamic calculations of these distributions presented in Berrill et al . [37] We digitized the coloured online pictures Fig. 2d from Berrill et al . [37] where two-dimensional spatial distributions of the electron density and small-signal gain at the time delay of 202 ps after the peak of the main prepulse are shown. In our calculations, we used the distribution of the electron density n e ( x , y ) obtained in this way without any changes. As for the gain distribution G ( x , y ), we used only the spatial profile g ( x , y ) and left G 0 as a fitted parameter because the absolute value of the gain obtained in Berrill et al . [37] does not exactly match the plasma used in our experiments. The second fitted parameter in our calculations was the saturation coefficient β . To adjust the parameters, we solved equation (1) that describes the amplification of seeded beam in a plasma amplifier. Varying G 0 and β parameters, as well as X-ray intensity at the input of the amplifier, we sought to achieve consistency between the calculated and experimental energy characteristics of our X-ray amplifier [26] . Coincidence has been achieved at β ~670 nJ cm −2 , gain coefficient G 0 ~36 cm −1 and the energy of the seeded beam W 0 ~770 nJ. Comparison of the theoretically calculated saturation curve with the experimental data from Nishikino et al . [26] is shown in Fig. 4c . It is seen that there is good agreement of the theoretical curve and the experimental data in the entire range of output amplifier energy. To ensure with greater certainty that our theory correctly describes the amplification of an injected pulse in the plasma amplifier, we calculated the angular spectrum of the output radiation for the selected above plasma parameters. The idea was to compare the calculated beam divergence, which is determined by the angular spectrum, with the experimentally measured divergence. The angular spectrum is shown in Fig. 4d . The beam divergence over x and y axes calculated as the full width at half-maximum was found to be ~2.4 × 0.6 mrad 2 . This is in full accordance with the experimentally measured beam divergence estimated from the beam image profile presented in Fig. 2a . Agreement of calculated and experimentally measured energies, as well as angular characteristics of the amplified radiation, verifies the adequacy of the proposed theoretical model. Besides, the obtained agreement shows that the chosen spatial distributions of the electron density and small-signal gain correctly describe optical properties of our plasma. The adjusted n e ( x , y ) and G ( x , y ) distributions are shown in Fig. 4a . For calculation of the mirage radiation, equations (2) and (3) were numerically integrated. The results of such simulations are presented in Fig. 4e , showing the appearance of a virtual X-ray point source in the centre of the plasma amplifier. Its location coincides, to within measurement errors, with its supposed position obtained by processing the experimentally observed fringes. Figure 4e shows the intensity profile of the virtual source beam at the output of the plasma and Fig. 4f shows its x−z cross-section inside the plasma. It is seen that the virtual source is well formed and is close to a point one with a waist diameter of ~2.5 μm. We can see a slight tilt of the beam to the z axis equal to ~1 mrad in the vicinity of the waist. This tilt is caused by the presence of an electron density gradient in the x direction, which leads to deflection of radiation towards the lower electron density. The above results demonstrate the formation of a mirage in a typical plasma with very complex profile. Both refraction and diffraction processes were taken into account. The additional information about the properties of X-ray mirage formation is given in Supplementary Discussion . The obtained results strongly support the hypothesis that was put forward earlier, about the formation in a plasma amplifier of a coherent virtual point source of X-rays phased with the radiation of the oscillator. We have shown that the discovered phenomenon can be interpreted as the first observation of the mirage phenomenon in the X-ray spectral region. The mirages were always associated with visible light ( Fig. 1 , inset) and has never been observed in X-ray range. Indeed, the appearance of a mirage in the X-ray range is extremely difficult because of low gradients of the refractive indexes of conventional media at these frequencies. Wilhelm Röntgen shortly after his opening of X-rays noted that the specificity of X-ray optics is that refractive index of all materials is close to 1. Obviously, the latter property practically eliminates the possibility of mirage formation in the X-ray range using conventional materials. In this sense, the laser-induced plasma is an absolutely unique medium. We have found the equation describing the mirage formation and have shown that a mirage can be coherent and can occur in the form of a coherent point source. The developed theory of X-ray mirages has a more general meaning. It adequately describes both refraction and diffraction phenomena accompanying the process of amplification. So, it allows for more accurate calculations of X-ray plasma amplifiers than the ray-tracing technique. We also believe that the theory could be successfully used for the optical range, in particular, for simulation of light-amplification processes in amplifying laser modules. There are various possibilities that the X-ray mirage phenomenon can be useful for further development of modern X-ray science and technology, for example, for generation of adaptively controlled phased X-ray beams, which could be applied to X-ray interferometry and tomography. Also, this effect can stimulate the further development of multistage X-ray lasers using laser-induced plasma as an active medium, because it changes the understanding of amplification of the X-ray pulses in the amplifying modules. Formation of the interference patterns themselves could be an effective method of diagnostics of plasma X-ray lasers, including the coherence degree of output radiation of such lasers. Obtained results have already demonstrated the effectiveness of this technique for the estimation of such plasma parameters as spatial profiles of the electron density and a gain coefficient. Experiment details The experiments were conducted with the SXRL laser [26] , [27] . The output pulse was generated with the nickel-like Ag plasma media using the oscillator-amplifier configuration shown schematically in Fig. 1 . Thin silver foils for the oscillator and the amplifier were pumped, respectively, with the line-focused travelling wave laser pulses with the proper timing for the effective amplification. A part of the SXRL beam from the oscillator was amplified in the plasma used as an amplifier. Emission spectrum corresponded to 4 d –4 p transition of a nickel-like Ag ion at 13.9 nm wavelength. The SXRL pulse after the amplifier had a bandwidth narrower than 10 −4 and a pulse duration of ~7 ps. The SXRL system worked in 0.1 Hz repetition regime with the typical output energy of the order of 300 nJ. Numerical simulations As already noted, the elaborated theory of the mirage and the mirage equation itself are written for an arbitrary-extended optically inhomogeneous amplifying medium, in particular, for any spatial distribution of n e ( x , y , z ) and G ( x , y , z ) of the plasma. For the solution of the whole problem, that is, for calculation of mirage radiation at the output of the plasma and for finding the position and shape of the virtual source in a particular physical situation, it is enough to numerically integrate equations (2 and 3) for given n e ( x , y ) and G ( x , y ). To do this, we rewrite the original equation (2) as: where and the complex amplitude of an incident field A inc ( x , y , z ) is considered to be given and the complex amplitude of X-ray mirage A M ( x , y , z )=0 at z =0. In our opinion, the most effective numerical method for solving such an equation is the split-step method [39] , which we applied for our calculations. For numerical solution of this parabolic equation, we used a rectangular grid of N x × N y elements with the spatial step sizes Δ x and Δ y in the x and y directions correspondingly. Decomposition of the total field into two fields, A M ( x , y , z ) and A inc ( x , y , z ), has allowed us to have a limited area where A M ( x , y , z ) is non-zero and also allowed to use the periodic boundary conditions of the split-step method. In numerical calculations, we used a diffraction limited Gaussian beam A G ( x , y , z )= as an incident radiation A inc ( x , y , z ). As equation (3) is a special case of equation (2), we used the same numerical procedure for its solution. The calculation scheme is graphically shown in Supplementary Fig. S3 . For the main calculations, we used the computational volume of 65 × 68 × 6,000 μm 3 size with 640 × 670 elements in x − y computational grid. The number of steps along z axis was 670. For the calculations according to the simplified model, described in Supplementary Discussion , the numbers were 200 × 200 × 6,000, 1,024 × 1,024 and 1,024 correspondingly. How to cite this article: Magnitskiy, S. et al . Observation and theory of X-ray mirages. Nat. Commun. 4:1936 doi: 10.1038/ncomms2923 (2013).